Predatory cannibalism inDrosophila melanogasterlarvae Hunting live prey is risky and thought to require specialized adaptations. Therefore, observations of predatory cannibalism in otherwise non-carnivorous animals raise questions about its function, adaptive significance and evolutionary potential. Here we document predatory cannibalism on larger conspecifics in Drosophila melanogaster larvae and address its evolutionary significance. We found that under crowded laboratory conditions younger larvae regularly attack and consume ‘wandering-stage’ conspecifics, forming aggregations mediated by chemical cues from the attacked victim. Nutrition gained this way can be significant: an exclusively cannibalistic diet was sufficient for normal development from eggs to fertile adults. Cannibalistic diet also induced plasticity of larval mouth parts. Finally, during 118 generations of experimental evolution, replicated populations maintained under larval malnutrition evolved enhanced propensity towards cannibalism. These results suggest that, at least under laboratory conditions, predation on conspecifics in Drosophila is a functional, adaptive behaviour, which can rapidly evolve in response to nutritional conditions. Predatory cannibalism, that is, killing conspecific in order to consume them, is arguably the ultimate selfish act. Although it can sometimes function to eliminate competitors [1] , [2] or be the price of mating [3] , it is usually a means of supplementing nutrition [4] , [5] , [6] , [7] . Cannibalism has important ecological consequences for population dynamics and stability, interspecific trophic interactions as well as pathogen transmission and epidemiology [8] , [9] , [10] . For predatory animals, cannibalism is a straightforward extension of diet and many predators include conspecifics among their prey [4] , [11] , [12] . A broader range of taxa engage in egg cannibalism, facilitated by the small relative size, immobility and defencelessness of eggs [2] , [6] , [13] , [14] , [15] , or in predation on much smaller juvenile conspecifics [8] , [11] . In contrast, herbivores or detritivores are presumably poorly equipped to hunt live conspecifics of size similar to (or larger than) themselves: lacking the morphological and behavioural adaptations of predators, they would be inefficient as hunters and risk injury by the victim defending itself [8] , [16] . Yet, instances of such predatory cannibalism have been reported in a number of otherwise non-carnivorous species, including insects [8] , [15] , [17] , [18] , [19] , [20] . These observations raise a number of questions. Is predatory cannibalism in herbivores or detritivores an aberrant or opportunistic outcome of chance encounters between potential cannibals and vulnerable victims, or do the cannibals take time from their normal foraging in order to hunt? Are specialized predatory behaviours, not used while feeding on normal food, involved in cannibalism? Does cannibalism have an adaptive value, that is, contribute to the Darwinian fitness, and if so, under what circumstances? Do populations harbour genetic variation for the propensity to cannibalism, allowing it to evolve in response to changing conditions? Affirmative answers to those questions would point to ecological importance of conspecific predation in non-carnivorous species and its potential significance in the evolutionary transition from herbivory or detritivory to a predatory lifestyle [20] . Data from diverse species provide partial answers to the above questions [8] . For example, in some anuran tadpoles cannibalism is mediated by morphological plasticity [21] , [22] and chemical cues [13] , and has an adaptive value in terms of nutrition and reduction of future competition [2] . In highly gregarious locusts and crickets cannibalism is an important source of protein and salts, which allows the cannibals to survive longer and migrate farther; cannibalism avoidance is an important factor driving their mass migrations [5] , [7] . The rapid response to artificial selection for reduced incidence of intraspecific predation in Spodoptera caterpillars [23] demonstrates that it is a heritable trait with substantial genetic variation. Although its benefits are unclear, cannibalism in Spodoptera carries a cost in terms of disease transmission [24] . Nonetheless, a comprehensive study of predatory cannibalism has been hindered by its apparent absence in genetically tractable model species. In this paper, we describe predation on conspecifics in Drosophila melanogaster larvae, and use it to address some of the above questions. In contrast to most other cases of cannibalism, cannibalism in Drosophila larvae involves attacks on victims larger than the cannibals. Using quantitative assays, we show below that, at least under laboratory conditions, this predatory cannibalism in D. melanogaster occurs regularly, involves specific behavioural responses to potential victims, is associated with phenotypic plasticity of the mouth parts and can improve survival, whereas the propensity to cannibalism is genetically variable and rapidly evolves in response to nutritional conditions. These results suggest that larval cannibalism in fruit flies is an adaptive behaviour that may contribute to Darwinian fitness under conditions of malnutrition. Drosophila larvae can be efficient predators on conspecifics We observed that, in mixed-age high-density laboratory cultures of D. melanogaster , younger (1st, 2nd and early 3rd instar) larvae regularly leave the food medium and crawl on the wall of the culture bottle, where they ‘track’ and attack large ‘wandering-stage’ 3rd instar larvae as the latter slow down to pupate ( Fig. 1a , Supplementary Movie 1 ). This behaviour was observed in several D. melanogaster strains of diverse origin: CantonS (an inbred laboratory strain), for R and for s (inbred strains carrying different alleles of the foraging gene [25] ), Valais and Fribourg (outbred populations derived from nature in Switzerland in 2006 and 2008, respectively), as well as in six selected and six control populations described below. By repeatedly rasping with their mouth hooks the attackers often managed to break the victim’s cuticle ( Fig. 1b , Supplementary Movie 2 ) and burrow into its body ( Fig. 1c ). Once wounded by the initial attackers, the victim attracted more attackers ( Fig. 1d , Supplementary Movie 3 ) and was typically consumed within 1–2 h. This collective cannibalistic behaviour possibly facilitates the overpowering of victims larger in size than the cannibals ( Supplementary Movie 1 ). 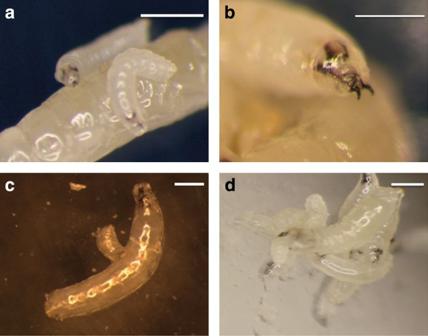Figure 1: Predatory cannibalistic behaviour inD. melanogasterlarvae. (a) First instar larvae attacking a wandering third-instar larva (see alsoSupplementary Movie 1). (b) A second instar larvae bares its mouth hooks to strike at the victim’s cuticle (see alsoSupplementary Movie 2). (c) First (or early second) instar larva burrowing into the flesh of a wandering larva. (d) Group cannibalism of a third-instar larvae by younger larvae on the walls of a culture bottle (see alsoSupplementary Movie 3). Scale bar=~0.5 mm. All photographs document spontaneous attacks initiated within culture bottles (that is, in the presence of food). Figure 1: Predatory cannibalistic behaviour in D. melanogaster larvae. ( a ) First instar larvae attacking a wandering third-instar larva (see also Supplementary Movie 1 ). ( b ) A second instar larvae bares its mouth hooks to strike at the victim’s cuticle (see also Supplementary Movie 2 ). ( c ) First (or early second) instar larva burrowing into the flesh of a wandering larva. ( d ) Group cannibalism of a third-instar larvae by younger larvae on the walls of a culture bottle (see also Supplementary Movie 3 ). Scale bar=~0.5 mm. All photographs document spontaneous attacks initiated within culture bottles (that is, in the presence of food). Full size image To quantify the efficiency of D. melanogaster larvae as predatory cannibals, we confronted, in vials with no food, groups of 25 younger larvae (potential cannibals, mostly at late 2nd instar, from two wild-type strains) with 10 healthy wandering-stage larvae (potential victims) carrying the sepia eye colour marker (to permit recognition of survivors). The ‘potential victims’ had already ceased feeding and would complete development even in the absence of food, but in the meantime were at the stage most vulnerable to cannibalism. These potential sepia victims suffered 35–40% mortality in the presence of the younger wild-type larvae ( Fig. 2a , ‘young’); in contrast, only about 8–10% sepia larvae failed to survive when confronted with 25 wandering-stage wild-type larvae that had already ceased feeding ( Fig. 2a , ‘wander’) or when maintained alone ( Fig. 2a ‘none’). In the absence of competition for food and with unlimited access to moisture (provided by agar), this difference in mortality of the potential victims ( F 1,12 =43.1, P <0.0001) was mostly or entirely the result of cannibalism by the younger larvae; indeed, many cases of cannibalism were observed in the experimental vials. Similar surplus mortality in the presence of potential cannibals was observed when the number of potential victims was increased to 25 to match the number of potential cannibals ( Fig. 2b ; F 1,12 =13.4, P =0.0032). The number of dead sepia larvae attributable to cannibalism (that is, the difference between the number of dead sepia larvae when confronted with younger versus wandering wild-types) was not affected by the number of sepia larvae ( sepia number × wild-type stage interaction, F 1, 6 =2.14, P =0.16). (The apparent marginally significant effect of wandering Valais larvae compared with sepia alone (‘none’) in Fig. 2b might reflect competition for pupation sites ( Fig. 2b ; F 1,9 =5.1, P =0.050), but would not be significant after correction for multiple comparisons.) Although rates of cannibalism would likely be lower in the presence of food, this experiment demonstrates that Drosophila larvae can be efficient predators of larger conspecifics. This indicates that cannibalism is not an aberrant outcome of chance encounters or that it only occurs on victims that are already weak or sick. 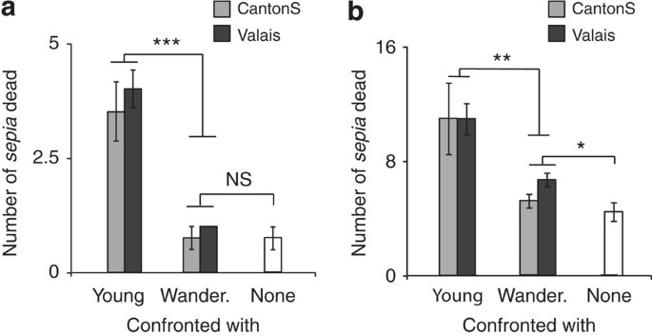Figure 2: A quantitative measure of cannibalistic behaviour. The number (mean±s.e.) of wanderingsepialarvae, out of 10 (a) or 25 (b), which failed to survive when confronted with 25 potential cannibals (92–94 h-old larvae; ‘young’) versus confronted with 25 wandering larvae (‘wander’), as well as in absence of antagonists (‘none’). The antagonists came from two wild-type strains (CantonS and Valais),N=4 vials per strain and treatment. The difference between the ‘young’ and ‘wander’ treatments estimates the effect of cannibalism; ***P<0.001, **P<0.01, *P=0.05. Figure 2: A quantitative measure of cannibalistic behaviour. The number (mean±s.e.) of wandering sepia larvae, out of 10 ( a ) or 25 ( b ), which failed to survive when confronted with 25 potential cannibals (92–94 h-old larvae; ‘young’) versus confronted with 25 wandering larvae (‘wander’), as well as in absence of antagonists (‘none’). The antagonists came from two wild-type strains (CantonS and Valais), N =4 vials per strain and treatment. The difference between the ‘young’ and ‘wander’ treatments estimates the effect of cannibalism; *** P <0.001, ** P <0.01, * P =0.05. Full size image Cannibalistic aggregations are mediated by chemical cues The ability to seek and detect prey is an essential adaptation for an efficient predator. We observed that in culture vials larvae gathered around on-going acts of cannibalism ( Fig. 1d , Supplementary Movie 3 ) and hypothesized that this aggregation was mediated by attraction to chemical cues released from victims injured in the attack. To test this hypothesis, we studied the movements of groups of 92–94 h-old larvae (counted from egg laying) on an agar plate containing one potential victim (wandering-stage) larva injured by pricking with a 0.15-mm needle (mimicking an injured victim of cannibalism) and one uninjured larva (both immobilized; Fig. 3a ). Placed initially at the centre, the larvae preferentially moved into the half of the plate containing the injured victim ( Fig. 3b ) and gradually many congregated in the vicinity (within 5 mm radius) of the victim ( Fig. 3c ); most victims were at least partially consumed. Instances of attacks on the immobilised uninjured larva were observed in some plates after the injured victim was consumed (~2 h later). The larvae used in this assay were well-fed (see Methods). In a separate assay, we found that larvae deprived of dietary protein (yeast and cornmeal) 24 h before assay congregated around the injured victim faster than those reared on standard food until the assay ( Fig. 3d ). This suggests that the motivation for cannibalism increases under protein deprivation. Attraction to injured victims was also observed when larvae were tested singly rather than in a group ( Fig. 3e ) and when the victims were of the same age as the test larvae ( Fig. 3f ). 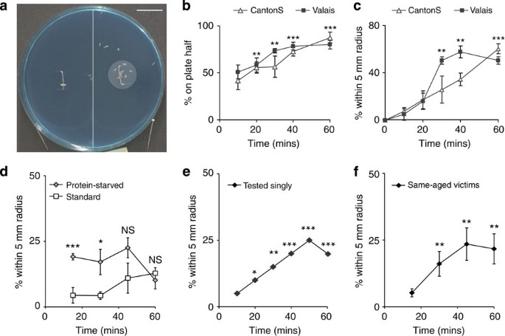Figure 3: Attraction to injured conspecifics. (a) The agar plate used to quantify larval attraction to injured versus uninjured conspecific victims, both immobilized with staple pins (scale bar=10 mm). At the beginning of the assay, the larvae were placed at the midline of the plate (highlighted line), equidistant from both victims. (b) Percentage (mean±s.e.) of larvae of two wild-type strains present on the half of the plate containing the injured victim and (c) within 5 mm radius of the injured victim (highlighted circular zone in panel a) as a function time since being released (N=4 plates with 20 larvae per strain). (d) Percentage (mean±s.e.) of larvae that were either protein-starved or reared on standard diet within 5 mm radius of the injured victim (N=4 plates of 20 larvae). (e) Attraction to injured conspecific in larvae tested singly: the percentage of larvae within 5 mm of the injured victim (N=20). (f) Attraction to injured victim similar in age to the test larvae (92–94 h): mean (±s.e.) percentage of test larvae observed within 5 mm of the injured victim;N=8 plates with 20 test larvae. In panels (d–f) only larvae of the Valais strain were used. In panels (b,c,e,f) the significance refers to null hypothesis that the proportion of test larvae within the target area (plate half or 5 mm radius) equals the proportion expected under random distribution (see Methods); in (b,c) the less significant of the twoP-values for two strains is indicated. In (d) the treatments were compared for each time point with at-test on arcsine-square-root-transformed proportions. *P<0.05, **P<0.01, ***P<0.001. Figure 3: Attraction to injured conspecifics. ( a ) The agar plate used to quantify larval attraction to injured versus uninjured conspecific victims, both immobilized with staple pins (scale bar=10 mm). At the beginning of the assay, the larvae were placed at the midline of the plate (highlighted line), equidistant from both victims. ( b ) Percentage (mean±s.e.) of larvae of two wild-type strains present on the half of the plate containing the injured victim and ( c ) within 5 mm radius of the injured victim (highlighted circular zone in panel a) as a function time since being released ( N =4 plates with 20 larvae per strain). ( d ) Percentage (mean±s.e.) of larvae that were either protein-starved or reared on standard diet within 5 mm radius of the injured victim ( N =4 plates of 20 larvae). ( e ) Attraction to injured conspecific in larvae tested singly: the percentage of larvae within 5 mm of the injured victim ( N =20). (f) Attraction to injured victim similar in age to the test larvae (92–94 h): mean (±s.e.) percentage of test larvae observed within 5 mm of the injured victim; N =8 plates with 20 test larvae. In panels ( d – f ) only larvae of the Valais strain were used. In panels ( b , c , e , f ) the significance refers to null hypothesis that the proportion of test larvae within the target area (plate half or 5 mm radius) equals the proportion expected under random distribution (see Methods); in ( b , c ) the less significant of the two P -values for two strains is indicated. In ( d ) the treatments were compared for each time point with a t -test on arcsine-square-root-transformed proportions. * P <0.05, ** P <0.01, *** P <0.001. Full size image These results suggest that cues released by attacked victims are perceived by other potential cannibals, which are roaming nearby, mediating the gregarious nature of cannibalism, which we observed on the walls of culture vials. Volatile cues would be less accessible to larvae engaged in normal feeding within the food substrate, but observations suggest that they can still find injured victims attractive at a close range and feed on them even in the presence of ample fresh food ( Supplementary Movie 4 ). Cannibalistic behaviour evolves under nutritional stress Finding widespread cannibalism in Drosophila larvae raises the question of the evolutionary advantage of the behaviour. If nutrition gained from the victim is the main benefit to the cannibals then populations frequently exposed to food shortage should evolve a greater heritable propensity towards cannibalism. We addressed this hypothesis with experimental evolution [26] , taking advantage of six experimentally evolved populations (‘selected’ populations) maintained for 118 generations on a poor-quality larval food and six control populations derived from the same base stock but maintained on standard food [27] , [28] . We compared their cannibalistic tendencies using the two quantitative assays described above. First, we found that 92–94 h-old selected larvae inflicted almost twice as high mortality than control larvae on healthy wandering sepia victims when confined with them in the absence of food ( Fig. 4a ; F 1,10 =12.7, P =0.005). Second, larvae from the selected populations aggregated significantly faster around experimentally injured victims ( Fig. 4b ; difference in slopes F 1,10 =5.8, P =0.037). Both these differences are heritable; because the tested selected and control larvae and their parents were raised on standard food before these assays, the effect of individual experience or maternal environment can be excluded. Therefore, as a result of being exposed to chronic larval malnutrition over many generations, the selected populations evolved to be more efficient hunters of uninjured conspecifics and better at locating already injured victims. These results support the notion that predatory cannibalism can be adaptive under nutritional stress, at least under laboratory conditions. They also demonstrate that there is enough genetic variation that allows a greater propensity for cannibalism to evolve within a short evolutionary time. 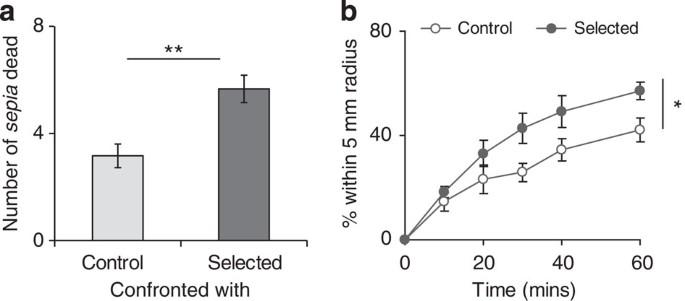Figure 4: Experimental evolution of propensity towards cannibalism. (a) The number (mean±s.e.) of wanderingsepialarvae (out of 10) which failed to survive when confronted with 92–94 h-old larvae from six populations selected for malnutrition tolerance and six control populations. **P=0.005, nested ANOVA (populations within treatments). (b) Attraction to injured victims (quantified as inFig. 2d) in control and selected populations, *P=0.037, nested ANOVA on regression slopes (see Methods). In both panels, the symbols are means±s.e. based on variation among replicate populations;N=6 populations × 4 replicates each per treatment. Figure 4: Experimental evolution of propensity towards cannibalism. ( a ) The number (mean±s.e.) of wandering sepia larvae (out of 10) which failed to survive when confronted with 92–94 h-old larvae from six populations selected for malnutrition tolerance and six control populations. ** P =0.005, nested ANOVA (populations within treatments). ( b ) Attraction to injured victims (quantified as in Fig. 2d ) in control and selected populations, * P =0.037, nested ANOVA on regression slopes (see Methods). In both panels, the symbols are means±s.e. based on variation among replicate populations; N =6 populations × 4 replicates each per treatment. Full size image Cannibalism is sufficient for survival The potential adaptive value of the cannibalistic behaviour in the context of food deprivation would be particularly evident if larvae could complete their entire development by cannibalizing other larvae [16] . To verify this, we reared Drosophila from egg to adult on an exclusively cannibalistic diet consisting of live but injured third-instar victims (three or six victims per 20 larvae per day). The larvae fed readily on the victims and a substantial proportion completed their development to adulthood ( Fig. 5a ). Even though this proportion of survivors was markedly smaller than the 80–90% typically observed on standard food, the fact that survival doubled when six rather than three victims per day were offered ( Fig. 5a ) shows that survival was more limited by the quantity than the quality of cannibalistic diet. The egg-to-adult developmental time of these survivors ( Fig. 5b ) was considerably longer than the 11–12 days typically observed in our laboratory on standard food [29] , and their adult weight was about half of that of flies raised on standard food ( Fig. 5c ). Even though the fecundity of adults raised on the cannibalistic diet was only half of that of flies raised on standard diet, they were capable of producing viable and fertile offspring ( Fig. 5d ). Altogether, the life history parameters of flies raised on the cannibalistic diet were similar to those observed on the poor-quality (diluted) cornmeal-sugar-yeast food medium used in our laboratory [29] . Thus, although a diet consisting entirely of conspecifics is certainly not optimal for D. melanogaster larvae, nutrition gained through cannibalism may be life-saving under extreme food shortage. As all three larval instars must feed for development to be completed [30] , this assay additionally confirms that all three larval instars are capable of cannibalism, at least if the victim is already injured. 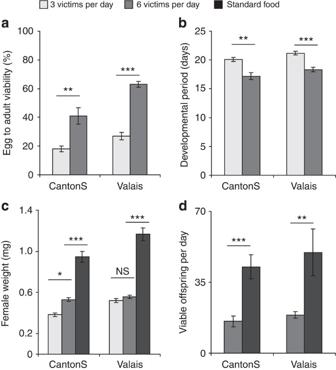Figure 5: Drosophila can successfully develop on a strictly cannibalistic diet. (a) Egg to adult viability and (b) developmental period of twoD. melanogasterstrains on different amounts of cannibalistic diet (three or six victims per day per vial); mean (±s.e.),N=5 vials with initially 20 eggs each. (c) Fresh weight of adult females reared on cannibalistic diet, compared with females raised on the standard diet;N=5 vials (2–6 females per vial). (d) Daily production of offspring surviving to adulthood by parents raised on cannibalistic diet versus standard food (the offspring were all raised on standard food);N=5 pairs. *P<0.05, **P<0.01, ***P<0.001,t-test. Figure 5: Drosophila can successfully develop on a strictly cannibalistic diet. ( a ) Egg to adult viability and ( b ) developmental period of two D. melanogaster strains on different amounts of cannibalistic diet (three or six victims per day per vial); mean (±s.e. ), N =5 vials with initially 20 eggs each. ( c ) Fresh weight of adult females reared on cannibalistic diet, compared with females raised on the standard diet; N =5 vials (2–6 females per vial). ( d ) Daily production of offspring surviving to adulthood by parents raised on cannibalistic diet versus standard food (the offspring were all raised on standard food); N =5 pairs. * P <0.05, ** P <0.01, *** P <0.001, t -test. Full size image Cannibalistic diet induces mouthpart plasticity Mouth parts of many animals show adaptive developmental plasticity in response to diet [31] , including spectacular differences between cannibalistic and non-cannibalistic siblings reported from amphibian tadpoles [21] , [32] . In D. melanogaster , a pair of mouth hooks are the main structure used for locomotion and feeding [30] . These mouth hooks are transitory hard chitin structures formed de novo at every moult. Each mouth hook is lined with teeth, which are used for food mastication [30] , but our observations show that they also have a key role in breaking the victim’s cuticle during a cannibalistic attack ( Supplementary Movie 2 ) and grating its flesh ( Supplementary Movie 5 ). Therefore, we examined the mouth hooks of larvae for plastic responses to cannibalistic diet. We found that third-instar larvae (staged morphologically [30] ) raised from egg on a strictly cannibalistic diet had about 20% more teeth than larvae reared on the standard food ( Fig. 6a–c ; F 1,36 =68.3, P <0.0001). To exclude that this is a consequence of generally poor nutrition we also examined the mouth hooks of larvae raised on the poor-quality food medium, which has similar effects on developmental time and adult size as the cannibalistic diet (see above). Larvae raised on the poor food had only slightly more teeth than those on raised on standard food ( F 1,36 =7.6 , P <0.02) and still considerably fewer than those raised on the cannibalistic diet ( Fig. 6c ; F 1,36 =34.7, P <0.0001). The increase in number of teeth is thus apparently a plastic response specific to being reared on the cannibalistic diet. Testing directly that this plastic response is adaptive would require either a way of manipulating teeth number independently of cannibalistic experience, which is not currently possible, or an evolution experiment [26] . Nonetheless, analogous plastic response observed in amphibian larvae has been shown to facilitate cannibalism [21] . 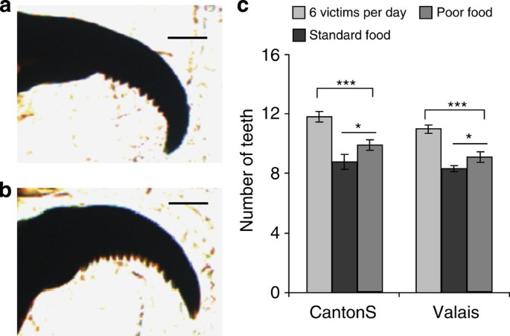Figure 6: Mouth hook plasticity in response to diet. Examples of mouth hooks of third-instar larvae reared on (a) standard and (b) cannibalistic diet; the teeth are visible on the inner (concave) edge (scale bar, 50 μm). (c) Tooth number of third-instar larvae of two strains reared on standard, poor and cannibalistic diets (6 victims per day), means (±s.e.),N=10 per strain and diet. *P<0.05, ***P<0.001; ANOVA. Figure 6: Mouth hook plasticity in response to diet. Examples of mouth hooks of third-instar larvae reared on ( a ) standard and ( b ) cannibalistic diet; the teeth are visible on the inner (concave) edge (scale bar, 50 μm). ( c ) Tooth number of third-instar larvae of two strains reared on standard, poor and cannibalistic diets (6 victims per day), means (±s.e. ), N =10 per strain and diet. * P <0.05, *** P <0.001; ANOVA. Full size image D. melanogaster are usually regarded as innocuous consumers of decomposing vegetable matter and the associated microbes. Nonetheless, larvae of a related species, Drosophila hydei , have been known to scavenge on carcasses of adult insects including conspecifics [33] , and at least one case of D. melanogaster larvae developing as parasites in a human has been reported [34] . Our study shows that the carnivorous taste of the larvae extends to active predation on conspecific larvae and could confer nutritional benefits, which could aid survival under nutritional stress, (in contrast to adult flies, which derive no measurable nutritional benefits from conspecific carcases [35] ). In contrast to most other cases of cannibalism [8] , [11] , in Drosophila most victims seem to belong to the stage with largest body mass, that is, pre-pupation wandering larvae, which are cannibalized by younger/smaller larvae. This ‘size-reversed’ cannibalism ceases to be a paradox once details of larval biology are taken into account. Wandering larvae have ceased feeding, and thus are unlikely candidates for cannibals themselves. Furthermore, larval mouth parts are not well adapted to predation, and breaking the victim’s cuticle requires prolonged rasping ( Supplementary Movie 2 ); therefore, attacking younger, agile larvae would be less likely to succeed. In contrast, even though wandering larvae can and do attempt to defend themselves by wriggling and striking back with their mouth hooks, the physiological processes leading to metamorphosis gradually make them virtually immobile [30] . This opens a window of vulnerability to cannibalism until their cuticle hardens into puparium. Nonetheless, larvae are also attracted to injured victims of similar age as themselves, suggesting that vulnerable victims of any stage may be targeted. Our observations indicate that cannibalism in D. melanogaster typically involves multiple larvae attacking the same victim, whereas experiments show that these cannibalistic aggregations are at least in part mediated by attraction to chemical cues from an injured victim. Recently reported visual attraction to larvae showing excessive wriggling [36] is possibly also motivated by cannibalism, as wriggling may indicate an on-going cannibalistic attack ( Supplementary Movie 1 ) or another injury. Although obviously not coordinated or truly cooperative, this ‘pack hunting’ presumably helps the attackers to overpower a larger victim. This would thus be another case of social facilitation, increasingly recognized as an important factor in Drosophila [33] , [37] , [38] . Our results indicate that cannibalism is promoted by nutritional stress. Spontaneous instances of cannibalism were mostly observed in crowded laboratory cultures, containing 15 or more larvae of different ages (originating from eggs laid over more than 24 h) per gram of food medium. Because under optimal conditions a fully developed larva contains about 11.5 J of energy and 0.13 mg protein [39] , the energy and protein content of the food medium (about 2,500 J and 10 mg protein per gram) should in theory be sufficient to support the development of those larvae. Nonetheless, after being used by the developing larvae for several days, the nutrients are partially depleted and contaminated with toxic metabolic waste products [40] , [41] . This deteriorating environment likely contributes to the incentive for larvae lagging in their development to leave the food medium and attempt to cannibalize wandering larvae, and numerous larvae were observed doing so. In contrast, few non-wandering larvae were seen leaving the medium in synchronized cultures at a standard density of 7–8 larvae per gram of food. Consistent with those observations, larvae deprived of protein for 24 h were more strongly attracted to injured victims, which points to their greater motivation for cannibalism. Furthermore, the experimental evolution of greater genetically based propensity towards cannibalism in populations maintained on poor larval food indicates that cannibalism is adaptive (that is, contributes to fitness) under malnutrition, at least under our laboratory conditions. Nonetheless, in our experimental assays even larvae well-fed until the assay showed attraction to injured conspecifics and successfully cannibalized non-injured wandering larvae within a few hours. Finally, we also observed larvae being attracted to and feeding on injured victims in the presence of ample fresh food ( Supplementary Movie 4 ). This suggests that cannibalism under laboratory conditions is not limited to larvae completely deprived of food; rather, its occurrence reflects an interaction between incentive and opportunity. While for larvae facing deteriorating nutritional conditions the incentive appears high enough to take the risk of pursuing the cannibalistic option away from the food, an opportunity offered by an easy victim is attractive even under optimal nutritional conditions. At this stage, we can only speculate about the potential significance of cannibalism in Drosophila in nature. Larval densities in nature are typically considerably lower than those in laboratory cultures; females are likely to avoid ovipositing on already crowded food if they have alternatives. Nonetheless, densities up to 8–12 (refs 42 , 43 ) adults emerging per gram of fruit in nature have been reported. There is also some evidence from several Drosophila species that the larvae can be nutritionally limited for growth and survival [42] , [43] , [44] , especially those hatching from eggs laid late, after the food patch has already been colonized for some time [45] . Desiccation or colonization of the food source by inedible and possibly toxic microorganisms [46] means that such latecomer larvae may face deterioration of their food source even if larval density is low; this would enhance the incentive to cannibalize conspecifics more advanced in their development. Furthermore, in addition to energy and protein, cannibalized conspecifics may be a source of limiting elements such as sodium [7] , which is scarce in fruits. However, even though cannibalism is facilitated in mixed-age groups, which commonly occur in nature [43] , [47] , the lower natural densities mean that encounters between larvae, and thus opportunities for cannibalism, are presumably much less frequent. Wandering larvae may also have greater chances of escape in nature than in laboratory cultures. If this reasoning is correct, the significance of cannibalism in nature would be limited more by opportunity than by incentive. Although these are speculations, several aspects of the behaviour suggest that predatory cannibalism is a normal component of the behavioural repertoire of fruit fly larvae and not merely an artefact of laboratory conditions. First, we observed cannibalism readily in strains of diverse origins. Second, larvae take time from normal feeding to track wandering victims outside of the food. Third, the cannibals often show persistence in their attack, continuing attempts to break the victim’s cuticle even though they are not getting an immediate food reward (for example, Supplementary Movie 2 ). Fourth, although we cannot demonstrate its adaptive nature, the phenotypic plasticity of mouth hooks in response to cannibalistic diet is reminiscent of mouth part plasticity in facultatively cannibalistic amphibian larvae [21] . Finally, in many species cues released by injured conspecifics represent a warning against potential danger (for example, predators) and induce avoidance [48] , [49] . In contrast, Drosophila larvae show attraction to injured conspecifics; similar behaviour in crickets is associated with cannibalism under natural conditions [7] . Thus, although direct evidence for its occurrence and ecological significance in nature is lacking, cannibalism in D. melanogaster has hallmarks of a specific, functional and coordinated behaviour, which is consistent with it having evolved by natural selection. The occurrence of cannibalism would change the view on competition within [50] and between Drosophila species [51] , [52] , [53] , hitherto thought to be solely based on scramble for food and tolerance to accumulated metabolic waste products [40] . We previously reported [50] that our selected populations exert greater negative effect on competitors than the controls; this study suggests that this could have been at least in part because of their enhanced cannibalism. Interestingly, Drosophila populations experimentally evolving under crowded conditions tend to diversify genetically into genotypes that develop rapidly but suffer high mortality and others that develop more slowly but are more tolerant to waste products and show better survival to adulthood [41] . Our study suggests that the slowly developing genotypes would have both an opportunity and an incentive to cannibalize the fast developers, thus potentially contributing to the higher mortality of the latter and thus to maintenance of the polymorphism. Competition involving direct aggression stabilizes population dynamics and may help maintain species diversity [1] , [9] , [12] . The ephemeral resources on which D. melanogaster larvae feed in nature are often utilized by a range of other species [51] , [52] , and the behaviours we describe here in the context of intraspecific predation could also be involved in predation on larvae of other species, that is, intraguild predation [54] . Our results suggest that species utilizing less protein-rich larval food sources may be expected to evolve a greater propensity towards both cannibalism and intraguild predation. These results also open a new perspective on the behavioural ecology and evolution of fruit flies and other non-carnivorous insects. Regular occurrence of cannibalism would alter the cost-benefit balance of larval aggregation observed in many herbivorous and detritivorous insects including Drosophila [55] . It would favour the evolution of defence and evasion behaviours [56] ; the wandering behaviour itself may have evolved as a strategy to evade cannibalism. It could promote the evolution of kin recognition to avoid cannibalizing siblings [57] . At longer evolutionary timescales, it could mediate evolutionary transitions to carnivory, explaining how a few fruit fly species (for example, D. simulivora ) became specialized predators [58] . Finally, even if cannibalism turns out to be of marginal significance for D. melanogaster in nature, finding regular cannibalistic behaviour in a model system opens the way for research on its sensory, neural and genetic basis. Fly stock and maintenance CantonS is an inbred strain maintained in the laboratory for several decades; Valais, an outbred strain derived from nature in Switzerland (2006); the sepia mutant strain was obtained from the Bloomington Stock Centre. Selected and control populations were all derived from the same base population: the six selected populations became adapted to larval malnutrition as a result of being maintained for 118 generations on highly diluted larval food; the six control populations were maintained on standard food (15 g agar, 30 g sucrose, 60 g glucose, 12.5 g dry yeast, 50 g cornmeal, 0.5 g MgSO 4 , 0.5 g CaCl 2 , 30 ml ethanol, 6 ml propionic acid and 1 g nipagin per litre of water) [27] , [28] . The poor larval food contained 25% of the amounts of sugars, yeast and cornmeal of the standard food. To minimize effects due to maternal environment, all strains were maintained on standard food at 25 °C for at least two generations before the assays. For all experimental data, as well as in the course of the 118 generations of laboratory evolution in selected and control populations, larval density was controlled by using 200–250 eggs per 30 ml of medium. However, some observations and filming of cannibalism were done on larvae from more crowded cultures; some of them were seeded with twice 200 eggs added on two consecutive days while in others adults were allowed to oviposit for 1–2 days without controlling egg density. Photography and filming The behaviours were video recorded and photographed using a Canon 7D DSLR camera mounted on a Leica stereo microscope. To document cases of natural attacks on initially uninjured victims, we identified cases of such an attack on the inner walls of culture bottle. The victims being attacked were carefully dislodged along with the cannibals and transferred on to an agar filled Petri plate for photography and filming. We also recorded cases of cannibalism provoked by offering the potential cannibals victims injured by pricking with a fine needle. In this case, the potential cannibal larvae were transferred to the petri plate 5–10 min before the victim to acclimatize. The videos were cut into smaller clips using iMovie HD software while the photographs were cropped using Windows Photo Editor. Quantifying the rate of cannibalism Wandering-stage larvae of the sepia mutant were used as potential victims, they were reared on standard food. Twenty-five 92–94 h-old wild-type larvae (potential cannibals), reared on standard food until the assay, were transferred together with 10 wandering sepia larvae (uninjured) to a 30-ml vial with the bottom covered with 2% agar (that is, without food). We subsequently recorded the number of emerging sepia adults in each vial. As a control to estimate the natural (cannibalism-unrelated) mortality of the wandering sepia larvae, we confined 10 wandering sepia with 25 wandering-stage wild-type larvae that have already ceased feeding. The proportion of sepia that died (that is, failed to emerge) was calculated for each vial (four vials per population). To compare the rate of cannibalism between the selected and control populations these proportions were arcsine-square-root-transformed and analysed with an analysis of variance (ANOVA), whereby the replicate populations were nested within the selected versus control regime. Assay of attraction to injured conspecifics To quantify attraction to injured potential victims, we presented groups of 20 larvae with a choice between an injured and an uninjured victim in 90 mm petri plates lined with 2% agar. The victims were wandering-stage larvae of sepia mutant immobilized with staple pins on the opposite sides of the plate; the injury was inflicted by pricking the larvae with a fine needle (0.15 mm thickness). The larvae whose behaviour was assayed were 92–94 h old counted from egg laying (their parents were allowed to oviposit for 2 h) and raised on standard food until the assay; they were thus well-fed. Based on other experiments at the same conditions, about 85% of these larvae should have been in the second instar and about 15% in the third instar (R.K. Vijendravarma, unpublished data). Twenty larvae were placed at the centre of the petri plate at time 0; the plates were photographed at 10, 20, 30, 40 and 60 min. The proportion of larvae within the plate half containing injured larvae and within 5 mm radius around the injured larvae at each time point were counted from the images using ImageJ ( http://rsbweb.nih.gov/ij/ ). Each plate was treated as one replicate. The proportions were arcsine-square root transformed before analysis. To verify that the larvae are actually attracted to the injured victim, we used Student’s t -distribution to test the null hypothesis that the observed proportions corresponds to the proportion expected under random distribution of larvae on the plate. This expected proportion was 0.5 for the half-plate, whereas for the 5 mm radius it was 0.01235 (the area within this radius, that is, 0.785 cm 2 divided by the entire area of the plate, that is, 63.6 cm 2 ). We also performed variants of this assay by maintaining tested larvae on a sugar agar medium for 24 h before the test (protein deprivation), using 92–94 h-old victims (instead of wandering-stage), and testing larvae singly instead of groups. In this last case, significance testing was based on binomial distribution with the expected proportion equal 0.01235, that is, the proportional size of the target area relative to the area of the whole plate, using two-tailed test. To compare the selected and control populations, attraction to injured victims was first quantified for each plate as the slope of regression of the proportion of larvae within 5 mm radius of the injured victim. The slopes were then compared using an ANOVA, with replicate populations treated as a random effect and nested within regime (that is, selected versus control). Development on exclusively cannibalistic diet Eggs of two wild-type strains (CantonS and Valais) were obtained by letting flies oviposit over 2 h on fruit jelly. The eggs were washed out of the jelly, rinsed with water and transferred in groups of 20 to a 30-ml vial with bottom covered with 2% agar. Nipagin (1 g l −1 ) was added to prevent microbial growth, including growth of yeast which might be a source of nutrition. To establish that there is indeed no nutrition available, in some vials nothing more was added; here, all hatched larvae died in their first instar. In other vials, soon after the eggs hatched and subsequently every 24 h either three or six injured third-instar sepia larvae were added to the vial. These victims had been raised on standard food, rinsed thoroughly with water to remove food medium residues, starved for 4–6 h to let them empty their guts, rinsed again and their cuticle was pierced at one spot on posterior half of the body with a fine needle (0.15 mm thickness). The number of emerging adults was recorded daily; these values were used to estimate the egg to adult viability and mean developmental time for each vial. We also measured the fresh weight of those flies (both sexes) at emergence. To study their fertility, adult virgin flies raised on the cannibalistic diet were transferred to standard food with live yeast supplement for 3 days. Subsequently, pairs were formed haphazardly and transferred every day for 5 days to a fresh vial with standard food. Eggs laid each day were counted; those laid on the 5th day were left in the vials to develop to give an estimate of egg-to-adult viability. Daily production of viable offspring was quantified as the mean number of eggs produced by each pair per day multiplied by viability. For comparison, we used the same approach to quantify the fertility of flies raised on standard diet. The treatments were compared with the t -test. Plasticity of mouth hook dentition Groups of 20 larvae were reared from egg on three different diets; a cannibalistic diet of six victims per day (as described above), on standard food and on poor food [27] . Mouth hooks of 10 third-instar (stage ascertained by the morphology of anterior spiracles) larvae per diet were dissected in saline and mounted on a glass slide in lactic acid: ethanol (6:5) and the teeth on each mouth hook were counted at × 50 magnification independently by two different researchers; in no case did the numbers obtained by the two researchers differ, indicating a perfect repeatability of the count. The average number of teeth on both mouth hooks was compared among diets using one-way ANOVA. How to cite this article: Vijendravarma, R. K. et al . Predatory cannibalism in Drosophila melanogaster larvae. Nat. Commun. 4:1789 doi: 10.1038/ncomms2744 (2013).